Probing the electronic structure at semiconductor surfaces using charge transport in nanomembranes The electrical properties of nanostructures are extremely sensitive to their surface condition. In very thin two-dimensional crystalline-semiconductor sheets, termed nanomembranes, the influence of the bulk is diminished, and the electrical conductance becomes exquisitely responsive to the structure of the surface and the type and density of defects there. Its understanding therefore requires a precise knowledge of the surface condition. Here we report measurements, using nanomembranes, that demonstrate direct charge transport through the π* band of the clean reconstructed Si(001) surface. We determine the charge carrier mobility in this band. These measurements, performed in ultra-high vacuum to create a truly clean surface, lay the foundation for a quantitative understanding of the role of extended or localized surface states, created by surface structure, defects or adsorbed atoms/molecules, in modifying charge transport through semiconductor nanostructures. Surfaces and interfaces strongly influence the electronic properties of semiconductor nanostructure [1] , [2] , [3] , [4] , [5] , [6] , [7] , [8] , and under some conditions they can become the dominant factor [3] . To investigate these influences quantitatively, a well-defined nanostructure is essential. In contrast to nanoparticles and grown nanowires, nanomembranes (NMs) provide the opportunity for such quantitative investigations, because they are two-dimensional crystalline sheets that can be fabricated using top-down methods, with precise surface orientations and sizes (lateral dimensions, thickness) and known doping levels. The free surfaces of NMs can be chemically modified in a homogeneous and predictable fashion, drawing on the long history of surface science. Finally, NMs can be easily simulated as a one-dimensional system, with all the benefits from size reduction remaining. In semiconductor nanomembrane systems, because the influence of the bulk is diminished, the electrical conductance reflects a high sensitivity to the surface. In a thin crystalline-semiconductor sheet, the simple existence of surfaces can significantly impact the bulk conductance of the sheet by providing states [3] , via a mechanism called surface transfer doping. But the surface may itself conduct, independent of the bulk, through extended electronic states at the surface that depend on the surface structure. This sensitivity of the electrical conductance to the surface suggests the possibility of using charge transport measurements on very thin sheets as a form of precision spectroscopy to obtain surface electronic structure information under well-defined conditions. The electronic structure at the surface is sensitive to atomic terminations and surface chemistries. Of course, in a thin-sheet geometry, one always has two interfaces. These can be made nominally identical for a free-standing NM [9] , but in practice the simpler and more relevant situation involves the nanomembrane resting on a host substrate, with an intervening dielectric layer. This dielectric layer allows use of the host substrate as a control gate. This back gate, which effectively changes the electrostatic potential in the NM, is a fundamental feature in the work we report here. It has many benefits. We demonstrate the feasibility of isolating the contributions of the two NM interfaces (the front free surface and the interface to the host) by varying the back-gate voltage as well as the NM thickness. A change in NM thickness modifies the coupling strength between the front free surface and the back gate, similar to the capacitance change from varying the dielectric-layer thickness in a conventional field-effect transistor (FET) configuration [10] . In fact, our device structures have much in common with standard Si-based FETs, except for the free, accessible front surface in our experiments and the use of four contacts plus the back gate. In the current measurements, the free surface is atomically clean, but that is not a requirement for general application of the method. Any changes [4] , [11] , [12] , [13] in the front surface act as an additional gate to counter or enhance the effect of the back gate. The NM bulk conductance is continuously tunable by the back-gate voltage and hence can be made negligible relative to the surface contribution. Through this approach we are able to extract fundamental properties of the electronic structure of clean (and subsequently chemically modifiable) silicon surfaces and, by extension, of many other crystalline-semiconductor or insulator systems in thin-sheet form. We can directly measure the surface conductance (for both an atomically clean surface and one that has been modified by adsorption or by structural damage), something of fundamental interest that is difficult to obtain by other means [14] . We demonstrate that we can determine reliably carrier mobilities in surface bands. We suggest that the combination of charge transport measurement with NMs to perform surface state spectroscopy can be applied to many materials systems beyond silicon, to extract the role of surfaces in modifying or controlling nanostructure electrical properties. Device structure and factors influencing the conductance For our experiments we use lightly doped silicon-on-insulator in the (001) configuration (SOI(001)) (Soitec, boron doping ~10 15 cm −3 ), thinned to the desired thickness, patterned into a van der Pauw configuration [15] , cleaned, and mounted on a specially designed sample holder that can be transferred into an ultra-high vacuum (UHV) chamber ( Fig. 1a ). The UHV environment (base pressure <1 × 10 −10 torr) enables preparation of samples with atomically clean surfaces, as well as surfaces with monolayers or submonolayers adsorbed in a controlled environment. Samples are introduced into vacuum immediately following an RCA (Radio Corporation of America) clean [16] and immersion in hydrofluoric acid (HF), which leaves the surface hydrogen (H) terminated [17] . The H is removed above ~500 °C. To produce the best structural surface order at the atomic level, we anneal the sample very briefly above 800 °C. The (2 × 1) clean-surface reconstruction indicative of good dimer row formation and therefore surface band formation is verified by observing the low-energy electron diffraction pattern. Samples are slightly miscut, by ±1° from the ‹001› direction. 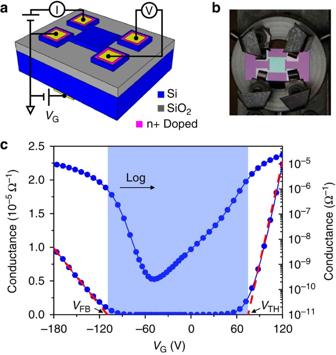Figure 1: Experimental setup and a conductance-voltage spectrum. (a) Schematic diagram of the van der Pauw measurement on a Si NM. The device mesa area is 4 × 4 mm2. The Si substrate serves as a back gate. (b) Image showing a sample mounted on the Mo sample holder. (c) Conductance as a function of back-gate voltageVGfor a 120-nm thick Si NM after hydrofluoric acid (HF) treatment. The data are plotted in linear (left) and log (right) scales. The flat-band voltageVFBand the threshold voltageVTHare extracted from linear extrapolations of the curve. Surface electrical information is determined from the low-conductance region (betweenVFBandVTH, shaded in blue). Figure 1: Experimental setup and a conductance-voltage spectrum. ( a ) Schematic diagram of the van der Pauw measurement on a Si NM. The device mesa area is 4 × 4 mm 2 . The Si substrate serves as a back gate. ( b ) Image showing a sample mounted on the Mo sample holder. ( c ) Conductance as a function of back-gate voltage V G for a 120-nm thick Si NM after hydrofluoric acid (HF) treatment. The data are plotted in linear (left) and log (right) scales. The flat-band voltage V FB and the threshold voltage V TH are extracted from linear extrapolations of the curve. Surface electrical information is determined from the low-conductance region (between V FB and V TH , shaded in blue). Full size image Figure 1c shows a typical conductance-gate voltage ( G-V G ) curve obtained from a Si NM (in this case H-covered), plotted in both linear and semi-log scale. In the linear-scale plot, both the electron inversion and hole accumulation regimes are visible, at the far right and far left ends of the graph, respectively. The turn-on voltages for these two channels, V TH (the threshold voltage) and V FB (the flat-band voltage), are extracted from linear extrapolations of the G-V G curve. The inversion and accumulation regions are well described by classical field-effect transistor theory [10] and are otherwise not the focus of this paper. In the depletion region, shaded light blue in Fig. 1c , surface/interface states and surface charge transport have deciding and competing roles. The plot on a log scale (upper curve) shows that slight changes in gate voltage lead to very large changes in the conductance. From these conductance characteristics we can extract surface electronic structure and determine mobilities of charge carriers moving in surface bands. 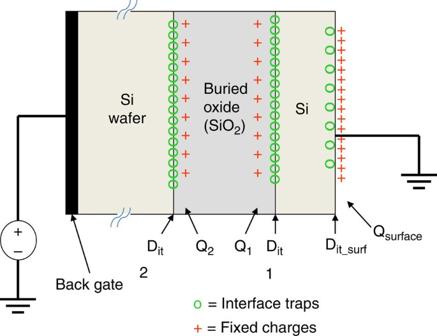Figure 2: Schematic diagram of a cross section of the structure considered in this work. The schematic cross section includes fixed charges, interface states and surface states. The Si handle wafer is much thicker than the top Si NM. The fixed charges influence the electrostatic field and thus modify the effective gate voltage. Figure 2 schematically illustrates the various factors that come into play in this measurement. In particular, at each interface and at the surface there exist fixed charges and localized states that can modify the electrostatic potential in the structure and can affect the resulting charge transport at the surface. Figure 2: Schematic diagram of a cross section of the structure considered in this work. The schematic cross section includes fixed charges, interface states and surface states. The Si handle wafer is much thicker than the top Si NM. The fixed charges influence the electrostatic field and thus modify the effective gate voltage. 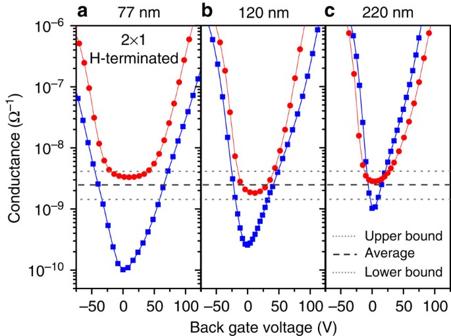Figure 3: Conductances for Si(001) NMs of different thicknesses and two surface conditions. Si(2 × 1) reconstructed surfaces (red circles) compared to the same NMs with adsorbed H (blue squares) for three different NM thicknesses: 77 nm (a), 120 nm (b) and 220 nm (c). The curves have been shifted along the voltage axis to put the minima at 0V. For clean reconstructed surfaces, there is always a flat region aroundGmin, in contrast to H-covered surfaces. The width of this region increases for thinner membranes. The horizontal dotted lines show the bounds of the conductance minima for all our clean-surface measurements. The average value is indicated by the dashed line and is 2.5 × 10−9Ohm−1. Full size image Conductance measurements and analysis Figure 3 shows the sheet conductance G as a function of normalized back-gate voltage for three thicknesses of Si(001) NMs with clean (2 × 1) reconstructed surfaces (red circles). By normalized we mean that the voltage is chosen as zero at the minimum conductance. The minimum value of conductance for the clean surface is independent of the sample thickness over the range considered here and for the bulk doping level of our samples. The shape near the minimum conductance for these NMs is essentially flat, with a broader minimum for thinner NMs, as expected from the dependence of capacitance on thickness. The horizontal dashed line at G min =2.5 × 10 −9 Ohm −1 is the average for all samples with thicknesses between 77 and 220 nm that we have investigated; the dotted lines at G min =2.5±1.0 × 10 −9 Ohm −1 show the maximum and minimum values of the minima in the measured conductance for these samples. Figure 3: Conductances for Si(001) NMs of different thicknesses and two surface conditions. Si(2 × 1) reconstructed surfaces (red circles) compared to the same NMs with adsorbed H (blue squares) for three different NM thicknesses: 77 nm ( a ), 120 nm ( b ) and 220 nm ( c ). The curves have been shifted along the voltage axis to put the minima at 0V. For clean reconstructed surfaces, there is always a flat region around G min , in contrast to H-covered surfaces. The width of this region increases for thinner membranes. The horizontal dotted lines show the bounds of the conductance minima for all our clean-surface measurements. The average value is indicated by the dashed line and is 2.5 × 10 −9 Ohm −1 . Full size image The clean-Si(001) (2 × 1) structure forms via dimerization [18] , [19] , creating an unoccupied surface π * band located 0.66 eV above the valence band edge, E V , and a filled surface π band 0.15 eV below E V [20] . Both bands are ~0.70 eV wide. The carrier concentration in the π * band depends on the precise Fermi level position at the surface, which is additionally influenced by defects on the Si(001)(2 × 1) surface [20] . Among the possible surface defects, type-C defects [21] , created by water molecules/OH- ions interacting with the Si surface [22] are the most prevalent; their density depends on sample preparation details, but it is not possible to eliminate them completely. As we show below, the conductance associated with the surface π * band formed by the dimers completely dominates the conductance-voltage curve around G min for the bulk doping levels and thicknesses of our NMs. Electrons are distributed among surface bands and surface defects and both are essential for understanding the data in Fig. 3 . The structure shown schematically in Fig. 2 is modelled as a one-dimensional system and the Poisson equation is solved numerically throughout its thickness to determine electrical properties of the surface. At each interface, the total amount of charge is calculated. The carrier distribution can be deduced from the simulation, and the membrane conductance is then calculated to fit the data, using as inputs the density of surface states and their position in energy. The above mentioned surface band positions [20] are used. 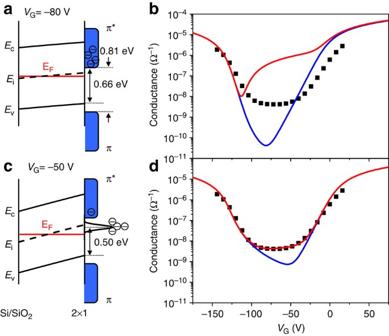Figure 4: Schematic diagrams of surface electronic structures and comparison of data and simulations for a 120-nm thick Si NM. (a,c): band diagrams without and with surface defect electronic structure. In (c) the peak indicates the energy position of the type-C defects. (b,d): corresponding calculations and experimental data. In (b) only surface bands are taken into consideration while in (d) type-C defects are added to the model. Black: data; blue curves: without surface charge mobility; red curves: with surface charge mobility. The π and π*band positions are taken from20. The type-C defects are described as a Gaussian distribution with a peak position 0.50 eV aboveEVand a full width at half maximum of 0.078 eV (3kBTat room temperature). The fitting parameters at the back Si/SiO2interface areDit=9.5 × 1011eV−1cm−2andQox=6.7 × 1011cm−2. The carrier mobility within the π*band is 45 cm2V−1s−1. Figure 4 shows comparisons of theory and experiment. The influence of the surface electronic structure on the NM conductance is first examined without contributions from surface defects ( Fig. 4a ). The π band makes essentially no contribution over the entire V G sweep, because the minimum separation of E F and the top of the π band is ~0.35 eV. On the other hand, the π * band effectively exchanges carriers with the SiNM bulk [3] . In Fig. 4b , the blue curve shows the NM conductance if charges in the π * band have zero mobility, that is, the surface band acts simply as a parking lot for charges. Even with zero mobility, the surface band has a large impact on the conductance; however, for zero mobility the simulated conductance has, for all reasonable values of surface band energy positions, a minimum that is two orders of magnitude lower than our experimental G min . Figure 4: Schematic diagrams of surface electronic structures and comparison of data and simulations for a 120-nm thick Si NM. ( a , c ): band diagrams without and with surface defect electronic structure. In ( c ) the peak indicates the energy position of the type-C defects. ( b , d ): corresponding calculations and experimental data. In ( b ) only surface bands are taken into consideration while in ( d ) type-C defects are added to the model. Black: data; blue curves: without surface charge mobility; red curves: with surface charge mobility. The π and π * band positions are taken from [20] . The type-C defects are described as a Gaussian distribution with a peak position 0.50 eV above E V and a full width at half maximum of 0.078 eV (3 k B T at room temperature). The fitting parameters at the back Si/SiO 2 interface are D it =9.5 × 10 11 eV −1 cm −2 and Q ox =6.7 × 10 11 cm −2 . The carrier mobility within the π * band is 45 cm 2 V −1 s −1 . Full size image To explain the relatively high minimum conductance in the data shown in Fig. 4 , a parallel conduction channel more conductive than several × 10 −9 Ohm −1 must exist. By adding a mobility for those electrons residing in the surface band, we are able to reduce the deep minimum to match that of the data. However, a surface band with non-zero mobility does not by itself reproduce the flat bottom observed in the measured conductance curve. The reason is that the surface band conductance changes in tandem with changes in the concentration of carriers in the surface band, which is effectively tuned by the back gate. The flat minimum in conductance is explained by the presence of defects at the surface that act to pin the Fermi level near but below the bottom of the π* band. This type of behaviour can be caused by type-C defects, which are always present (typically at a density of 1%) and pin the Fermi level at the surface [21] . Their influence on the band structure is shown schematically in Fig. 4c . Simulation results including the effect of type-C defects are shown in Fig. 4d , again with and without surface band conduction. With no surface band conduction, G min is still approximately one order of magnitude lower than our experimental value: in other words, a higher and constant density of charges in the π * band is insufficient to fit the data. Furthermore the curve still has a decidedly asymmetric shape, which is never observed experimentally. Thus, the charges in the π * band have to be able to move, and adding a direct surface band contribution to the total conductance (red curve) is essential to flatten out the bottom region. Simulations of the total conductance, that is, the NM bulk conductance plus the surface band conductance in the presence of surface Fermi level pinning, is plotted in Fig. 4d as the red curve. The calculated result shows a very good match to the experimental data. The essence of our argument is that the thickness independence of the conductance minimum as a function of back-gate voltage of our atomically clean Si(001) NMs is an indication that in the depletion region the clean-surface conductance dominates for all NM thicknesses up to at least 220 nm. We argue that this conductance is caused by the clean-surface reconstruction via the establishment of surface bands. We can examine this proposition by passivating the surface and eliminating the surface reconstruction and thus the surface bands. The most direct way is to repeat the measurements with H on the surface. The H-covered Si(001) surface is terminated primarily with dihydrides [17] and is quite disordered [23] . The blue curves in Fig. 3 show data for H-terminated samples: they display a minimum in conductance that becomes deeper as the NM becomes thinner. The absence of the surface conduction channel in the H-terminated surface results in the differences between the red and the blue curves in Fig. 3 . Any surface conduction in a H-terminated surface must be less than the deepest minimum, 10 −10 Ohm −1 , one to two orders of magnitude smaller than the surface conductance of the clean surface. Details on the H-terminated Si NMs will be presented elsewhere. We have therefore experimentally established that the clean-surface π * bands contain mobile charges. As mentioned above, the fits to the clean-surface measurements require a charge carrier mobility in the π * band. We obtain values from 10 to 70 cm 2 V −1 s −1 . Although it is clear that the charges must be mobile, the values of surface charge carrier mobility are considerably smaller than the Si bulk carrier mobility at room temperature. The corresponding mean free path calculated using the classical Drude model is ~10 nm, a value that approaches the mean separation of atomic-height steps (terrace widths) on our Si(001) surfaces (1° miscut). The dimer row directions on adjacent terraces are orthogonal. 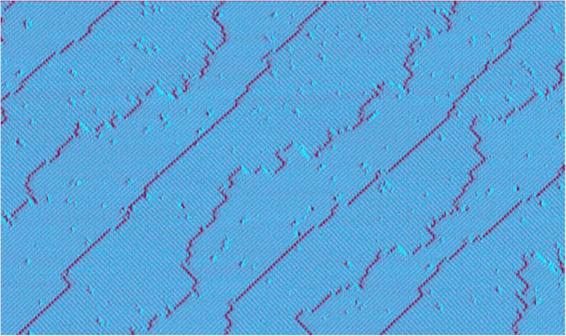Figure 5: Scanning tunneling micrograph of a Si(001) surface miscut toward ‹110› by ~1°, giving mean terrace widths of ~10 nm. Image diagonal: ~100 nm. The image is shown in derivative mode to accentuate steps, dimer rows and surface defects. The surface steps down from upper left. Image courtesy Brian Swartzentruber. Figure 5 shows a representative scanning tunnelling micrograph of a slightly miscut Si(001) surface that illustrates these points [24] . Scattering mechanisms for charges in the surface bands are so far not explored, but it is reasonable to expect that steps will scatter charges. The charge density in the surface band is also low, but can be modified with temperature and the density of surface point defects. Figure 5: Scanning tunneling micrograph of a Si(001) surface miscut toward ‹110› by ~1°, giving mean terrace widths of ~10 nm. Image diagonal: ~100 nm. The image is shown in derivative mode to accentuate steps, dimer rows and surface defects. The surface steps down from upper left. Image courtesy Brian Swartzentruber. Full size image Prior efforts have been made to probe surface conduction, using instead of thin sheets poorly conducting bulk substrates, which intrinsically have low conductance, but obtaining reliable results is experimentally very challenging [14] . Measurements on bulk semiconductors are dominated by other parallel conduction channels, including bulk conduction and conduction through the space charge region, as the surface conductance is typically several orders of magnitude smaller. Microscopic probes, such as the scanning tunneling microscope [25] , [26] , [27] and microscopic cantilevers [28] , [29] , have been utilized to make surface conductance measurements, but only one study uses thin sheets of Si [30] , as found in SOI. Because of a reduced penetration of electric field into the bulk, the use of smaller probe spacings maximizes the surface contribution to charge transport in measurements on bulk samples. Nevertheless, the surface conductance cannot be measured reliably using these methods and is likely overshadowed by charge transport through the charge depletion region. The measured surface conductance thus has a large uncertainty. Experimental results for the surface conductance in the more commonly investigated Si(111)-(7 × 7) surfaces span 5 orders of magnitude [14] , from 10 −3 to 10 −8 Ohm −1 . Additionally, the carrier occupation of the surface band must be estimated from other techniques, such as photoemission [31] . We are aware of only one surface conductance measurement performed on Si(001)(2 × 1) surfaces [30] , with a reported value on the order of 10 −6 Ohm −1 , three orders of magnitude higher than the result we report here. These measurements were performed with SOI of the SIMOX (separation by implantation of oxygen) type [32] . The surface conductance was determined as the difference between the total conductance of an atomically clean surface and an oxygen saturated one; however, without back gating, which was not possible because the buried oxide in SIMOX SOI is quite leaky. Therefore, the fixed oxide charge (see Fig. 2 ) could not be considered in the band model used to calculate the depletion region conductance. NMs allow measurement of surface charge transport because conduction through the NM bulk is already small. By preserving our oxide quality, we are able to add gate voltage into the measurement, allowing us to neutralize the effects of fixed oxide charge, which effectively acts as an additional gate voltage, and to reach the minimum total conductance in the depletion region. Moreover, by varying the NM thickness, effects arising from the front surface and the back interface can be separated. Thus, we can determine the Si/SiO 2 interface state density and the surface electron occupation at the same time. As mentioned, we directly extract the surface conductance of Si(001)(2 × 1) from the flat bottom region of the conductance-voltage spectra. From the carrier distribution required to fit the conductance, the charge carrier mobility in the surface band can be determined. An important component to our approach is to measure membranes with different thicknesses, as the free-surface effects scale reciprocally with the membrane thickness, while the bottom-interface effects do not. A consistent surface electrical model can be achieved for both H-terminated (Peng et al ., unpublished data) and clean (2 × 1) reconstructed surfaces for all three membrane thicknesses considered in our experiments. The back interface properties are essentially independent of membrane thickness. In summary, we have made conductance measurements in UHV on thin Si sheets (Si NMs). From the shape of conductance plots as a function of back-gate voltage, we conclude that electron transport must occur through the surface bands themselves. Simulations are able to reproduce the experimental results with high precision, and they allow an extraction of the surface band mobility, which for all samples is on the order of 50 cm 2 V −1 s −1 . The shape of the curves for the (2 × 1) surface termination indicates the presence of Fermi level pinning, which we attribute to type-C defects at the surface. The approach of combining nanometer-thick sheets with back-gated electrical transport measurements should be universal for investigating surface transport in semiconductor materials. Device fabrication The van der Pauw pattern (a mesa of dimensions 4 × 4 mm 2 ) in SOI(001) is fabricated using standard lithography and dry etched down to the buried oxide. The nominal doping of the substrate is p-type, N A ~10 15 cm −3 . Highly doped contacts are made to the layer through four square pads (see Fig. 1 , main text) that each are connected to the central mesa by a 500-μm wide and 500 μm long arm. The resulting contacts are expected to result in errors from the ideal (zero contact length) van der Pauw results of <1%. The contacts are intentionally doped with n-type spin-on-dopant (SOD, P-8545 from Honeywell) and annealed at 800 °C for 5 min using rapid thermal annealing. Secondary ion mass spectrometry reveals that this procedure results in degenerately doped Si within the top several tens of nanometres, sufficient for working contacts in both the electron and hole-operating regimes. The Si substrate is contacted and used as a back gate. Surface preparation The sample is cleaned in acetone and isopropanol, followed by a 15-min UV ozone treatment. It is then chemically cleaned using a standard RCA I procedure followed by an HF dip. Although HF treatment leaves the Si surface hydrophobic, a brief N 2 blow dry is necessary because of residual HF droplets left on the exposed SiO 2 region. The sample then is mounted onto a specially designed sample holder, which is transferred into the UHV chamber within <30 min after preparation. To prepare a clean surface, the sample is heated to 850 °C for 10 s by electron bombardment from the backside, followed by rapid cooling. This procedure is repeated several times until a sharp (2 × 1) low-energy electron diffraction pattern is observed. During heating the temperature is directly measured with an infrared pyrometer. The measurement on the clean reconstructed surface begins 45 min after the last heating cycle to let the sample cool. Electrical measurements For each back-gate voltage, eight four-probe measurements are made, from which we deduce the conductance per square using the standard van der Pauw formulas [15] . During the van der Pauw measurement, the electrical properties of the silicon template layer are nonuniform in the direction along the film thickness (see Fig. 2 of the main text). For example, at large backgate voltages an inversion layer is found at the back interface, while the surface band is at the top surface. By using the van der Pauw analysis, we implicitly assume the template layer is thin enough (220 nm or less) compared with its lateral dimensions (4 × 4 mm 2 ) that equilibrium between the front and the back interfaces is achieved over lateral length scales much smaller than the device dimensions. In other words, the sample is uniform laterally. To the extent that this assumption is incorrect, it will introduce errors in the correspondence between theory and experiment. How to cite this article: Peng, W. et al . Probing the electronic structure at semiconductor surfaces using charge transport in NMs. Nat. Commun. 4:1339 doi: 10.1038/ncomms2350 (2011).